Controlled multi-vinyl monomer homopolymerization through vinyl oligomer combination as a universal approach to hyperbranched architectures The three-dimensional structures of hyperbranched materials have made them attractive in many important applications. However, the preparation of hyperbranched materials remains challenging. The hyperbranched materials from addition polymerization have gained attention, but are still confined to only a low level of branching and often low yield. Moreover, the complication of synthesis only allows a few specialized monomers and inimers to be used. Here we report a ‘Vinyl Oligomer Combination’ strategy; a versatile approach that overcomes these difficulties and allows facile synthesis of highly branched polymeric materials from readily available multi-vinyl monomers, which have long been considered as formidable starting materials in addition polymerization. We report the alteration of the growth manner of polymerization by controlling the kinetic chain length, together with the manipulation of chain growth conditions, to achieve veritable hyperbranched materials, which possess nearly 70% branch ratios as well as numerous vinyl functional groups. Hyperbranched (HB) polymers have received much attention in scientific fields far beyond polymer science. They offer superior features such as low viscosity, good solubility and a high range of functionality. Moreover, their much simpler and more cost-effective synthesis mechanism [1] , [2] have allowed HB polymers to be considered as alternatives to dendrimers for emerging applications in a variety of fields, ranging from nano-building blocks, microelectronics and sensors to applications in drug delivery [3] , [4] , [5] . To date, polycondensation of AB n -type monomers still predominate in synthetic approaches to HB polymers [6] , [7] , but this approach suffers from poor control over the polymer structure. With the introduction of controlled/living polymerization, one of the most successful approaches is the self-condensing vinyl polymerization (SCVP) introduced by Fréchet [8] , [9] , [10] , [11] , [12] , [13] . Another approach is the copolymerization of a single vinyl monomer with a multi-vinyl monomer (MVM). It has been long recognized that without any particular precaution, such as low MVM concentration or dilute solution condition, this copolymerization leads to the formation of insoluble networks, as predicted by the Flory–Stockmayer (F–S) theory. The introduction of a chain transfer agent in this polymerization allowed the synthesis of various soluble highly branched polymers, thanks to the increase of primary chain concentration. This strategy, coined ‘Strathclyde synthesis’ [14] , was then enriched, thanks to living/controlled radical polymerization mechanisms. The so-called controlled radical crosslinking copolymerization methodology has enabled the synthesis of various branched polymers with very well-defined primary chain lengths [15] , [16] , [17] , [18] , [19] , [20] , [21] , [22] , [23] . However, only low proportions of MVM could be used to avoid gelation, which limits the formed polymers to a low branching degree. The soluble products cannot be HB polymers but only ‘highly’ branched ones. HB polymers can be defined as structures in which each monomer unit is either a branching unit or a potential branching unit. Resorting to controlled radical polymerization mechanisms, the only access up to now to such HB structures has been the aforementioned SCVP approach. However, this approach suffers from its lack of versatility as it implies tailor-synthesized inimers. In this contribution, we propose a new approach to the synthesis of HB polymers, based on the controlled radical homopolymerization of MVMs. This ‘Vinyl Oligomer Combination’ approach has allowed the successful fabrication of unprecedented HB polymer architectures with an extremely high branching density as well as numerous vinyl functional groups. This HB architecture consists purely of extremely short primary chains, which is fundamentally distinct from the architecture produced by any previous method (for example, ‘Strathclyde synthesis’, controlled radical crosslinking copolymerization and even SCVP). We provide solid evidence to demonstrate that it is possible to kinetically and statistically control and manipulate the HB structure in the homopolymerization of MVMs in a concentrated polymerization system. This new approach demonstrates great advantages for the synthesis of HB polymers for industrial applications, through its sheer simplicity, monomer possibilities (broad range of commercially available MVMs) and high yield. The control over the homopolymerization of MVMs has been long considered as an impossible task, as the F–S mean field theory predicted that the polymerization of MVM only lead to insoluble crosslinked materials even at low conversion [24] , [25] , [26] , [27] , [28] , [29] . Indeed, the inclusion of only small amounts of MVMs, if carried out in addition polymerizations, for example, free radical polymerization (FRP), will result in the formation of a macroscopic crosslinked network of MVMs. However, a deactivation-enhanced atom transfer radical polymerization (DE-ATRP) strategy can efficiently delay the gel point of the MVM homopolymerization up to 60% monomer conversion in a concentrated polymerization system [30] , [31] , [32] . By this approach, a novel three-dimensional ‘single cyclized’ architecture was formed attributable to the suppressed intermolecular reactions ( Fig. 1a ). This discovery prompted us to develop a new model that gives a significant supplementation to the classical F–S theory based on the space and instantaneous growth boundary concept [30] . Most importantly, this study subverted the traditional impression of MVMs reactions—‘uncontrolled and challenging’. Doors have now been opened for the design and manipulation of various polymer architectures from the homopolymerization of MVMs. 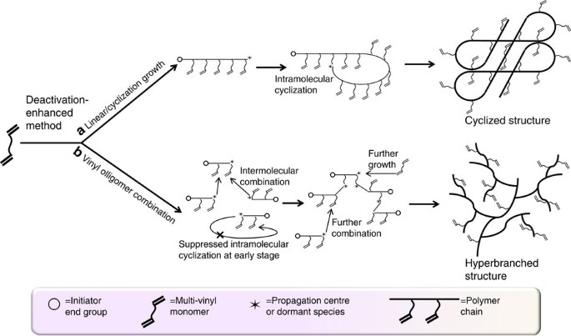Figure 1: Polymerization strategies leading to cyclized or HB structures. Homopolymerization of MVM via DE-ATRP with different strategies leading to either cyclized or HB structures. (a) Under the condition of a restricted growth boundary (small kinetic chain length), cyclized structures are formed through the strategy of intra-enhanced propagation. The intramolecular cyclization is enhanced owing to the high local/spatial vinyl concentration within the growth boundary. (b) HB structures are formed under the strategy of vinyl oligomer combination. The intermolecular reaction is facilitated from early reaction stages when numerous oligomers are formed and become the predominant species in the reaction system. In this situation, the intramolecular cyclization is suppressed owing to the small chain length during the linear growth period. Figure 1: Polymerization strategies leading to cyclized or HB structures. Homopolymerization of MVM via DE-ATRP with different strategies leading to either cyclized or HB structures. ( a ) Under the condition of a restricted growth boundary (small kinetic chain length), cyclized structures are formed through the strategy of intra-enhanced propagation. The intramolecular cyclization is enhanced owing to the high local/spatial vinyl concentration within the growth boundary. ( b ) HB structures are formed under the strategy of vinyl oligomer combination. The intermolecular reaction is facilitated from early reaction stages when numerous oligomers are formed and become the predominant species in the reaction system. In this situation, the intramolecular cyclization is suppressed owing to the small chain length during the linear growth period. Full size image It is well known that two types of reactions lead to the formation of crosslinks during crosslinking copolymerization or MVM homopolymerization: intramolecular crosslinking (cyclization), leading to the formation of ‘loops’ in the structure, and intermolecular crosslinking, leading to the increase of molecular weights through the formation of crosslinks between chains. As aforementioned, we already investigated the case of favoured intramolecular events during MVMs homopolymerization, leading to single-cyclized polymers [30] , [31] . This led us to ask a further question: if the intramolecular reaction can be enhanced by the suppression of intermolecular reactions (leading to a cyclized polymer structure), how can the intermolecular reaction be facilitated with the suppression of intramolecular reactions? Theoretically in this situation, a maximally HB structure should be possible. To achieve the HB structure, two critical parameters must be adhered to. The first is the low kinetic chain length that is the length that a growing chain reaches in a single active cycle. As reported before [32] , in situ DE-ATRP retains a large proportion of deactivated species (via Cu II ) and thus significantly decreases the kinetics chain length (ν=k p [M]/k de [Cu II ]). Using this strategy, it is possible to make the propagation rate of a polymer chain much slower than the deactivation rate, and thus minimize kinetics chain length to an extremely low level ( Supplementary Fig. S1 ). The second crucial premise is the high ratio of initiator to MVM. This will not only lead to extremely short primary chains but also will decrease the chance of intramolecular cyclization at the early reaction stage. In this study, we introduce a high initiator to divinyl monomer ratio at 1:2. We hypothesize that short linear chains or oligomers will form at the early stages of the reaction according to statistical prediction, and then large-scale intermolecular combination occurs at a later reaction stage when a certain concentration of oligomer chains is reached ( Fig. 1b ). Analysis of polymerization process Monitoring the homopolymerization of 1,3-butanediol diacrylate (BDA) via DE-ATRP by size exclusion chromatography (SEC) at regular time intervals during the reaction provides us with data that strongly support our proposed mechanism ( Fig. 2a ). It can be clearly seen that at first (within 1 h) the polymerization mixture consists mainly of monoadducts of monomer and initiator as well as a certain portion of oligomers. The more broadening of peaks at 2 h (PDI=1.6) and 3.5 h (PDI=3.7) suggests that the combination of lower molecular weight oligomers appears to be the major reaction pathway at the later stage. It is likely that at later stages of the reaction, with most of the monomer already consumed, the reaction conditions are more favourable for statistical branching rather than for linear growth. Vinyl conversion at 3.5 h reached 69% ( Table 1 , Supplementary Fig. S2 ) and the precipitated polymer possessed a branch ratio of 66% (the percentage of divinyl-consumed branched units in all of the constructive units, Supplementary Fig. S3a ), which is much higher than the previously reported MVM-derived polymers [30] , [31] , [32] , [33] . This high branch ratio indicates a highly branched structure formed from the enhanced intermolecular coupling rather than the traditional chain growth. 1 H NMR analysis during the reaction shows that the majority of combination events occur when the initiator is nearly exhausted. Gas chromatography (GC) was also performed to monitor composition evolution during the early period of polymerization [34] ( Supplementary Fig. S4 ). Monomer conversion at 0.5 h (32%) and 1 h (60%), calculated from GC, are approximately twice as high as the vinyl conversion (18% for 0.5 h and 34% for 1 h), which is in accordance with the assumption that the divinyl monomer are mainly consumed on one side instead of on both sides and very few of branched units are formed at the early period of the reaction. Mass spectroscopy was also performed for the 0.5 and 1 h samples to investigate the composition at the early period of reaction ( Fig. 3a ). It can be clearly seen that the polymerization mixture within 1 h consists mainly of monoadduct as well as a certain portion of oligomers, matching with the SEC results. The number gap between each major peak is exactly the molecular weight of BDA, which indicates that the molecular weight increases by 1 unit and the vinyl groups of the divinyl monomer are mainly consumed on one side instead of on both sides at the beginning period. A comparison experiment was performed with low initiator to monomer ratio (1:100). SEC traces show that the polymerization process also occurs in two distinct phases ( Fig. 2b ). At first, the polymer chains display an initial linear-like growth. The increase of molecular weight is linear with monomer conversion, and PDI remains low with unimodal molecular distribution. Then, only at much later stages of the polymerization process, chain combination occurs and is accompanied by the rapid increase in M w and PDI. However, a certain proportion of branched units (18%) is formed in the first phase of the reaction (5 h, PDI=1.3, vinyl conversion=9%, Table 1 , Supplementary Fig. S3b ), which provides evidence for the dominance of cyclization reactions occurring during the linear growth process at the begining of this comparison polymerization. 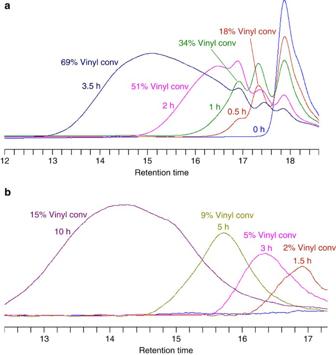Figure 2: Time dependence of the composition of the polymerization mixtures. Mixtures are monitored by SEC equipped with a refractive index (RI) detector, showing the different reaction pathways. (a) HB polyBDA, indicating that the divinyl monomer first underwent a large-scale linear oligomerization (<1 h) followed by oligomer combination (>1 h); (b) cyclized polyBDA, showing the unimodal peaks typically at initial stages (<5 h) and multimodal peaks appearing later (>5 h). Significant multimodality in the case of HB polyBDA, especially for low and moderate molar masses, is not observed in the case of single-cyclized polyBDA. This strongly supports the expected differences in terms of mechanism: in the case of single-cyclized polyBDA (almost exclusively intramolecular cyclization), the increase of molar masses is only owing to propagation, whereas in the case of HB, it is mainly owing to intermolecular combination. Figure 2: Time dependence of the composition of the polymerization mixtures. Mixtures are monitored by SEC equipped with a refractive index (RI) detector, showing the different reaction pathways. ( a ) HB polyBDA, indicating that the divinyl monomer first underwent a large-scale linear oligomerization (<1 h) followed by oligomer combination (>1 h); ( b ) cyclized polyBDA, showing the unimodal peaks typically at initial stages (<5 h) and multimodal peaks appearing later (>5 h). Significant multimodality in the case of HB polyBDA, especially for low and moderate molar masses, is not observed in the case of single-cyclized polyBDA. This strongly supports the expected differences in terms of mechanism: in the case of single-cyclized polyBDA (almost exclusively intramolecular cyclization), the increase of molar masses is only owing to propagation, whereas in the case of HB, it is mainly owing to intermolecular combination. Full size image Table 1 Polymerization conditions and molecular weight characteristics of the polymers with different structures. 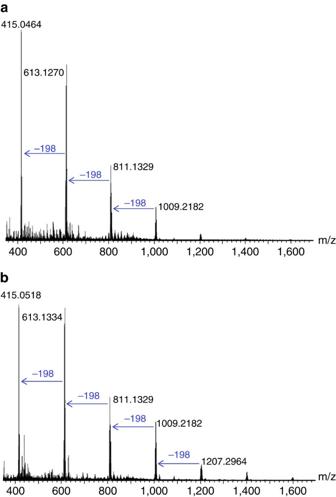Figure 3: Mass spectra of early stages of polymerization. Mass spectrum for the samples from early period of polymerization of HB polyBDA, showing the chemical composition within the polymerization system. (a) Mass spectrum of 0.5 h sample inFig. 2a; (b) mass spectrum of 1 h sample inFig. 2a. The number gap between each major peak is exactly the molecular weight of BDA, which indicates that the molecular weight increases by 1 monomer unit and the vinyl groups of the divinyl monomer are mainly consumed on one side instead of on both sides at the beginning period. Full size table Figure 3: Mass spectra of early stages of polymerization. Mass spectrum for the samples from early period of polymerization of HB polyBDA, showing the chemical composition within the polymerization system. ( a ) Mass spectrum of 0.5 h sample in Fig. 2a ; ( b ) mass spectrum of 1 h sample in Fig. 2a . The number gap between each major peak is exactly the molecular weight of BDA, which indicates that the molecular weight increases by 1 monomer unit and the vinyl groups of the divinyl monomer are mainly consumed on one side instead of on both sides at the beginning period. Full size image Universality Furthermore, we have demonstrated that this strategy to HB structures can be widely applied to the polymerization of a broad range of MVMs, including the derivatives of acrylate, methacrylate, styrene, and so on. Similar results were achieved with the homopolymerization of di(ethylene glycol) diacrylate (DEGDA), ethylene glycol dimethacrylate and divinylbenzene (DVB) ( Supplementary Table S1 , Supplementary Fig. S5 ). Degradation test To further prove that our proposed strategy leads to such a highly branched structure, a cleavable polymer was designed and prepared via in situ DE-ATRP from a degradable disulphide divinyl monomer (DSDA) [35] . Within the DSDA monomer is a disulphide bond that can be cleaved quickly under reducing conditions, thus allowing us to observe the degradation profile and hence determine if a hyperbranced structure (will be degraded into small units) or a cyclized structure (will ‘untie’ into a linear chain) is formed. In a similar fashion, the DSDA homopolymerization towards a HB structure was monitored by SEC as shown in Supplementary Fig. S6 , which presents a similar profile to that obtained for BDA. Vinyl conversion reached 74% at 10 h without gelation ( Table 2 , Supplementary Fig. S7 ). 1 H NMR spectra for purified HB polyDSDA (10 h, M w =30.9 kDa, PDI=5.0) are shown in Supplementary Fig. S8 . Recently, Armes and co-workers [36] developed a quantification method for the intramolecular cyclization by 1 H NMR spectrum analysis. However, this quantification method is not suitable for analysing this new polyDSDA polymers as the proton d (O– CH 2 –) overlaps with the proton k and the residue linear unit. Instead, by integration of the initiator end group (proton j and h) and that of the DSDA units (proton of e), we were able to calculate the ratio of initiator units to DSDA units. This ratio was calculated to be 1:1.9, which means that each primary chain consists of only ~1.9 DSDA units. This result proves that the HB polymer consisted of extremely short primary chains. Table 2 Polymerization conditions and molecular weight characteristics of the hyperbranched polyDSDA. Full size table It can be expected that the HB disulphide polymer, if combined by addition of primary vinyl oligomer, would degrade into oligomers when the intermolecular branch units are broken ( Fig. 4a ). The SEC result of the final disulphide polymer before and after degradation confirms our predicted result. The high molecular weight polymer chains were indeed degraded into small chains, and the molecular weight showed a very large reduction after degradation ( Fig. 4b , Supplementary Fig. S9 ). It can be noticed that the distribution of the cleavage product is broad and multimodal. The components consist of big portions of extremely small molecules and some oligomers. The degradation result provides a profound comparison to the very slight molecular weight reduction observed when the ‘single cyclized’ structure was degraded as previously reported [30] , [31] . It is clearly proved that the polymer prepared by the vinyl oligomer combination approach possessed a highly branched structure and that intermolecular combination reactions are the main contributor to the high branch ratio. 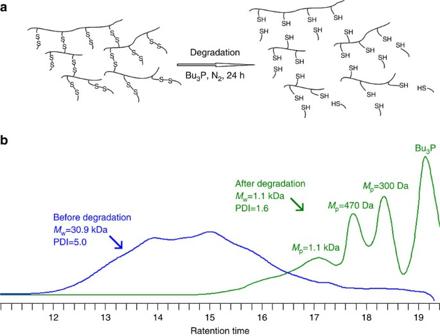Figure 4: Schematic representation and degradation of the disulphide polymer. (a) Schematic representation of the degradation that would occur from the disulphide polymer to linear primary chains by disulphide bond cleavage using reduction of tributylphosphine (Bu3P).Mwand hydrodynamic size of polymer chains will decrease significantly in branched polymers. (b) The SEC trace before and after cleavage of the HB polybis(2-acryloyl)oxyethyl disulphide (polyDSDA) synthesized by vinyl oligomer combination strategy (purified 10 h product inTable 2andSupplementary Fig. S6. After purification, theMwincreased from 21.5 to 30.9 kDa because the precipitation process removed parts of the molecules with low molar mass). The HB structure was proved by the substantial decrease in molecular weight and hydrodynamic size after cleavage. Figure 4: Schematic representation and degradation of the disulphide polymer. ( a ) Schematic representation of the degradation that would occur from the disulphide polymer to linear primary chains by disulphide bond cleavage using reduction of tributylphosphine (Bu 3 P). M w and hydrodynamic size of polymer chains will decrease significantly in branched polymers. ( b ) The SEC trace before and after cleavage of the HB polybis(2-acryloyl)oxyethyl disulphide (polyDSDA) synthesized by vinyl oligomer combination strategy (purified 10 h product in Table 2 and Supplementary Fig. S6 . After purification, the M w increased from 21.5 to 30.9 kDa because the precipitation process removed parts of the molecules with low molar mass). The HB structure was proved by the substantial decrease in molecular weight and hydrodynamic size after cleavage. Full size image With a deeper analysis of the reaction environments, it becomes less difficult to understand the factors that determine which reaction type will lead to different polymer architectures (as shown in Fig. 5 ). More specifically, three parameters, including the growth boundary (kinetic chain length), the chain dimension and the chain concentration, are all taken into account. A relatively small growth boundary, which depends on the kinetics chain length, strictly confines the small number of monomers added to an active centre and thus keeps the polymer chains growing in a limited space. In this way, unlike what happens in FRP, the formation of huge polymer chains and large-scale combination at the early reaction stages are avoided. Therefore, a small growth boundary, which can be achieved by in situ DE-ATRP, is the basic prerequisite for the formation of either the maximal HB structure or the ‘single cyclized’ structure. So under this condition of a small growth boundary, different chain dimensions and concentrations will lead to distinct reaction types. A low ratio of initiator to monomer would result in the formation of longer chains but with a lower chain concentration, which would no doubt increase the chance of intramolecular reactions due to the high local/spatial vinyl concentration within the growth boundary. Although the opportunity for intermolecular reactions can rise as the polymer chains grow, this probability at the early stage of reaction can be neglected because of the low chain concentration. That is why a ‘single cyclized’ polymer can form as the main product. However, in contrast, a high initiator concentration not only diminishes the chain dimension during the linear-growth phase and thus suppresses the intramolecular cyclization, but also it increases the chain concentration in the system so that pendent vinyl groups in one chain are more likely to fall into the growth boundary of another chain. After the monomers massively convert to short chains, the intermolecular combination increases and allows the formation of HB structures with a high density of branching and vinyl functional groups. 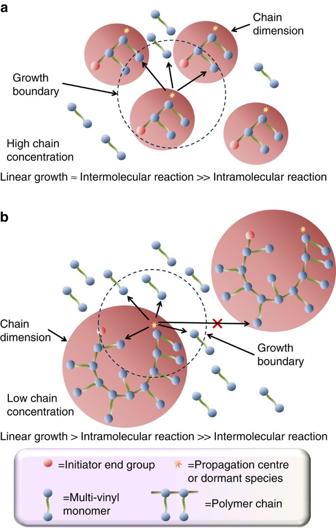Figure 5: Formation of different structures viain situDE-ATRP. (a) Formation of HB structure; (b) Formation of ‘single cyclized’ structure. Three parameters are considered: the growth boundary (dotted circle), chain dimension (red shaded part) and chain concentration. The growth boundary, which confines the possible number of vinyl groups reacted within its active lifetime during the propagation process, could change the selectivity of vinyl groups attacked by the propagation centre. The probability of intermolecular combination decreases with distance between an active propagation centre and another polymer chain, which is strongly dependent on the chain dimension and chain concentration. Figure 5: Formation of different structures via in situ DE-ATRP. ( a ) Formation of HB structure; ( b ) Formation of ‘single cyclized’ structure. Three parameters are considered: the growth boundary (dotted circle), chain dimension (red shaded part) and chain concentration. The growth boundary, which confines the possible number of vinyl groups reacted within its active lifetime during the propagation process, could change the selectivity of vinyl groups attacked by the propagation centre. The probability of intermolecular combination decreases with distance between an active propagation centre and another polymer chain, which is strongly dependent on the chain dimension and chain concentration. Full size image We demonstrated that MVM homopolymerization can be kinetically oriented so as to favour very different polymer architectures with two possible extreme topologies: either single-cyclized or HB polymers, that is, crosslinking consists exclusively of intramolecular or intermolecular reactions, respectively. Whereas the intermolecular formation would cause the number of primary chains per polymer molecule to increase, a cyclic substructure would result from the intramolecular reaction, thus called cyclization. It should be noted here that a network, which can be defined topologically by the existence of several paths between constitutional units through the structure, would necessarily imply both types of crosslinking reactions. In particular, it is important to distinguish HB structures presented in this work from nanogels [37] , which can be defined as swollen polymer networks with a size under 100 nm and can be therefore considered as soluble highly branched polymers too: the formation of nanogels implies a contribution of cyclizations, whereas HBs are achievable through intermolecular crosslinking only. Up to now, no analytical technique can provide a direct distinction between HB polymers and nanogels, which exhibit similar behaviours. The nature of the topology can be deduced from the combination of the analysis of the products with the knowledge of initial parameters, which directly impose key structural characteristics, such as the initial initiator concentration imposing the primary chains concentration, and so on. In the present contribution, even if intramolecular events cannot be totally ruled out (a few cyclization reactions may occur), the experimental conditions implemented clearly favour the formation of HB polymers. This is strongly supported by the SEC analyses of products prepared using the disulphide crosslinker: an important shift towards lower molecular weights is observed after cleavage (no significant modification is expected if intramolecular crosslinks are cleaved). A supplementary argument is the primary chain length, which is so short here that it excludes any significant contribution of cyclizations: if two primary chains are already linked through a crosslink, there are no more monomer units available to enable the formation of a second crosslink between them. In conclusion, it has been shown here that by using the kinetic control theory to manipulate chain growth conditions, we can design two clearly different polymer structures, including a veritable HB polymer with a high branch ratio of 66% and a large amount of vinyl functional groups. It can be foreseen that this new strategy for preparation of HB polymers could open up the field to the polymerization of a very wide range multifunctional vinyl monomers or combinations of comonomers in any proportion. We envisage that a broad range of new highly branched functional polymers with novel properties will be obtained from a variety of economical and structurally special MVMs, which will have important applications in a variety of different fields. Materials BDA (98%), acryloyl chloride (≥97%) and 2-hydroxyethyl disulphide (90%) were purchased from Sigma-Aldrich. Bis(2-acryloyl)oxyethyl disulphide (disulphide-based diacrylate, DSDA, ≥95%) was synthesized according to literature. DEGDA (75%), ethylene glycol dimethacrylate (EGDMA, 98%) and DVB (80%) was purchased from Sigma-Aldrich. The ethyl 2-bromoisobutyrate (EBriB, 98%, Aldrich) was used as the initiator. Pentamethyldiethylenetriamine (PMDETA, 99%, Aldrich), Triethylamine (TEA, 99%, Aldrich), copper (II) bromide (CuBr 2 , 97%, Aldrich), L -ascorbic acid (AA, 99%, Aldrich), tributylphosphine (Bu 3 P 97% Aldrich), D -Chloroform (99.8%, Aldrich), 2-butanone (HPLC grade, Aldrich), toluene (HPLC grade, Aldrich), tetrahydrofuran (THF, HPLC grade, Aldrich), n -hexane (ACS reagent grade, Aldrich), diethyl ether (ACS reagent grade, Aldrich) and dichloromethane (DCM, ACS reagent grade, Aldrich) were used as received. Preparation and purification of the bis(2-acryloyl)oxyethyl disulphide monomer 2-Hydroxyethyl disulphide (9.79 ml) and TEA (22.25 ml) were added in a two-necked round bottom flask, with THF (200 mol) as solvent. Acryloyl chloride (25.8 ml) was then added dropwise under the argon protection. The flask was sealed and the mixture was stirred in an ice bath for 24 h. The by-produced salt was removed by filtering under reduced pressure. The reaction mixture was redissolved in DCM and extracted with sodium carbonate aqueous solution (Na 2 CO 3 , 0.1 M), then purified by basic alumina column with DCM as eluents. The obtained product of bis(2-acryloyl)oxyethyl disulphide was determined by 1 H NMR in CDCl 3 : 2.84 p.p.m. t (4H), 4.45 p.p.m. t (4H), 5.80 p.p.m. d (2H), 6.05 p.p.m. q (2H) and 6.43 p.p.m. d (2H). Preparation of HB polyBDA BDA (20 mmol, 2 equiv), 2-butanone (8.5 ml), EBriB (10 mmol, 1 equiv), CuBr 2 (0.5 mmol, 0.05 equiv) and PMDETA (0.5 mmol, 0.05 equiv) was added into the flask, and oxygen was removed by bubbling argon through the solutions for 20 min at room temperature. AA (0.15 mmol, 0.015 equiv) was carefully transferred into the flask under an argon blanket. The solution was stirred at 800 r.p.m. and the polymerization was conducted at 60 °C in an oil bath for the desired reaction time. Preparation of HB polyDEGDA DEGDA (20 mmol, 2 equiv), 2-butanone (8.5 ml), EBriB (10 mmol, 1 equiv), CuBr 2 (0.5 mmol, 0.05 equiv) and PMDETA (0.5 mmol, 0.05 equiv) was added into the flask and oxygen was removed by bubbling argon through the solutions for 20 min at room temperature. AA (0.15 mmol, 0.015 equiv) was carefully transferred into the flask under an argon blanket. The solution was stirred at 800 r.p.m. and the polymerization was conducted at 60 °C in an oil bath for the desired reaction time. Preparation of HB polyEGDMA Ethylene glycol dimethacrylate (EGDMA, 20 mmol, 2 equiv), 2-butanone (8.5 ml), EBriB (10 mmol, 1 equiv), CuBr 2 (0.5 mmol, 0.05 equiv) and PMDETA (0.5 mmol, 0.05 equiv) was added into the flask and oxygen was removed by bubbling argon through the solutions for 20 min at room temperature. AA (0.0375, mmol, 0.00375 equiv) was carefully transferred into the flask under an argon blanket. The solution was stirred at 800 r.p.m. and the polymerization was conducted at 60 °C in an oil bath for the desired reaction time. Preparation of HB polyDVB DVB (20 mmol, 2 equiv), toluene (8.5 ml), EBriB (10 mmol, 1 equiv), CuBr 2 (0.5 mmol, 0.05 equiv) and PMDETA (0.5 mmol, 0.05 equiv) was added into the flask and oxygen was removed by bubbling argon through the solutions for 20 min at room temperature. AA (0.25 mmol, 0.025 equiv) was carefully transferred into the flask under an argon blanket. The solution was stirred at 800 r.p.m. and the polymerization was conducted at 90 °C in an oil bath for the desired reaction time. Preparation of HB polyDSDA Bis(2-acryloyl)oxyethyl disulphide (disulphide-based diacrylate, DSDA, 20 mmol, 2 equiv), 2-butanone (8.5 ml), EBriB (10 mmol, 1 equiv), CuBr 2 (0.5 mmol, 0.05 equiv) and PMDETA (0.5 mmol, 0.05 equiv) was added into the flask and oxygen was removed by bubbling argon through the solutions for 20 min at room temperature. AA (0.15 mmol, 0.015 equiv) was carefully transferred into the flask under an argon blanket. The solution was stirred at 800 r.p.m. and the polymerization was conducted at 60 °C in an oil bath for the desired reaction time. Preparation of cyclized polyBDA BDA (20 mmol, 100 equiv), 2-butanone (8.5 ml), EBriB (0.2 mmol, 1 equiv), CuBr 2 (0.5 mmol, 2.5 equiv) and PMDETA (0.5 mmol, 2.5 equiv) was added into the flask and oxygen was removed by bubbling argon through the solutions for 20 min at room temperature. AA (0.15 mmol, 0.015 equiv) was carefully transferred into the flask under an argon blanket. The solution was stirred at 800 r.p.m. and the polymerization was conducted at 60 °C in an oil bath for the desired reaction time. Purification of HB and cyclized polymer The experiment was stopped by opening the flask and exposing the catalyst to air. Samples taken from reaction at different reaction time points were diluted with butanone and precipitated into a large excess of mixed solvent of hexane and diethyl ether (1:1) to remove monomer. The precipitated mixture was redissolved in tetrahydrofuran followed by passing through a silica column to remove the residual copper. The product solution was evaporated in vacuum at room temperature for 2 h and collected for further analysis. The procedure for the cleavage of polyDSDA About 0.05 g of purified polyDSDA was dissolved in 2 ml of THF followed by adding 30 μl of Bu 3 P. The mixture was stirred at room temperature for 2 h and collected for further analysis. Polymerization of methyl acrylate Methyl acrylate (40 mmol, 4 equiv), 2-butanone (8.5 ml), EBriB (10 mmol, 1 equiv), CuBr 2 (0.5 mmol, 0.05 equiv) and PMDETA (0.5 mmol, 0.05 equiv) was added into the flask and oxygen was removed by bubbling argon through the solutions for 20 min at room temperature. AA (0.15 mmol, 0.015 equiv) was carefully transferred into the flask under an argon blanket. The solution was stirred at 800 r.p.m. and the polymerization was conducted at 60 °C in an oil bath for the desired reaction time. SEC characterizations of HB and cyclized polymer Weight average molecular weight ( M w ), number average molecular weight ( M n ) and polydispersity ( M w / M n ) were obtained by SEC (Varian 920-LC) equipped with a RI detector. The columns (30 cm PL gel Mixed-C, two in series) were eluted using THF and calibrated using a series of 12 near-monodisperse PMMA standards ( M p from 690–1,944,000 g mol −1 ). The polymers were analysed in THF at a concentration of 5.0 mg ml −1 . All calibrations and analysis were performed at 40 °C and a flow rate of 1 ml min −1 . 1 H NMR characterizations of HB and cyclized polymer 1 H NMR analysis was carried out on a S4 300 MHz Bruker NMR with JEOL Delta v5.0.1 processing software. The chemical shifts were referenced to the lock chloroform (7.26 p.p.m.). GC characterization GC analysis was carried out with a Varien 3900 chromatograph using an RTx-5 crossbound 5% diphenyl/95% dimethyl polysiloxane (15 m × 0.25 mm × 0.25 μm) column. The oven temperature is set to 200 °C with the heating rate of 30 °C min −1 . Mass spectrometry characterization Electrospray ionization mass spectra were acquired using a Waters LCT Premier XE time-of-flight mass spectrometer equipped with electrospray ionization source (Water Corp., Milford, MA). Samples were dissolved in (specify solvent) and introduced into the instrument via a Water Corp. Alliance 2795 separations module at a rate of 20 μl min −1 using a syringe pump and a polyetheretherketone capillary line. The heated capillary temperature was 250 °C and the spray voltage was 5 kV. How to cite this article: Zhao, T. et al. Controlled multi-vinyl monomer homopolymerization through vinyl oligomer combination as a universal approach to hyperbranched architectures. Nat. Commun. 4:1873 doi: 10.1038/ncomms2887 (2013).